In silicomethod for modelling metabolism and gene product expression at genome scale Transcription and translation use raw materials and energy generated metabolically to create the macromolecular machinery responsible for all cellular functions, including metabolism. A biochemically accurate model of molecular biology and metabolism will facilitate comprehensive and quantitative computations of an organism's molecular constitution as a function of genetic and environmental parameters. Here we formulate a model of metabolism and macromolecular expression. Prototyping it using the simple microorganism Thermotoga maritima , we show our model accurately simulates variations in cellular composition and gene expression. Moreover, through in silico comparative transcriptomics, the model allows the discovery of new regulons and improving the genome and transcription unit annotations. Our method presents a framework for investigating molecular biology and cellular physiology in silico and may allow quantitative interpretation of multi-omics data sets in the context of an integrated biochemical description of an organism. A goal of systems biology is to provide comprehensive biochemical descriptions of organisms that are amenable to mathematical enquiry [1] . These models may then be used to investigate fundamental biological questions [1] , guide industrial strain design [2] and provide a systems perspective for analysis of the expanding ocean of omics data [3] . Over the past decade, there has been steady progress in developing genome-scale models of metabolism (M-Models) for basic research and industrial applications [4] , [5] , [6] . M-Models are stoichiometric representations of the enzymatic and spontaneous biochemical reactions associated with an organism's metabolic network at the genome scale; however, M-Models do not quantitatively describe gene expression ( Fig. 1a ). The lack of an explicit representation for enzyme production precludes quantitative interpretation of omics data and can result in biologically implausible predictions [7] , [8] . Because M-Models do not contain chemical representations of transcription and translation, to date, it has only been possible to use omics data as ad hoc constraints for enzyme activities [9] , [10] , [11] , [12] . 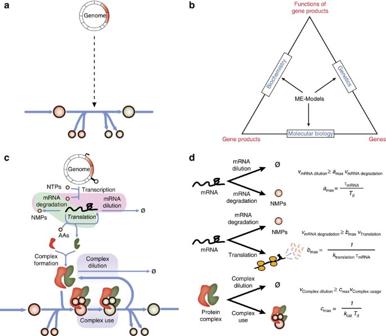Figure 1: Genome-scale modelling of metabolism and expression. (a) Modern stoichiometric models of metabolism (M-models) relate genetic loci to their encoded functions through causal Boolean relationships. The gene and its functions are either present or absent. The dashed arrow signifies incomplete and/or uncertain causal knowledge, whereas blue arrows signify mechanistic coverage. (b) ME-Models provide links between the biological sciences. With an integrated model of metabolism and macromolecular expression, it is possible to explore the relationships between gene products, genetic perturbations and gene functions in the context of cellular physiology. (c) Models of metabolism and expression (ME-Models) explicitly account for the genotype–phenotype relationship with biochemical representations of transcriptional and translational processes. This facilitates quantitative modelling of the relation between genome content, gene expression and cellular physiology. (d) When simulating cellular physiology, the transcriptional, translational and enzymatic activities are coupled to doubling time (Td) using constraints that limit transcription and translation rates as well as enzyme efficiency.τmRNA, mRNA half-life;kcat, catalytic turnover constant;ktranslation, translation rate;ν, reaction flux. Figure 1: Genome-scale modelling of metabolism and expression. ( a ) Modern stoichiometric models of metabolism (M-models) relate genetic loci to their encoded functions through causal Boolean relationships. The gene and its functions are either present or absent. The dashed arrow signifies incomplete and/or uncertain causal knowledge, whereas blue arrows signify mechanistic coverage. ( b ) ME-Models provide links between the biological sciences. With an integrated model of metabolism and macromolecular expression, it is possible to explore the relationships between gene products, genetic perturbations and gene functions in the context of cellular physiology. ( c ) Models of metabolism and expression (ME-Models) explicitly account for the genotype–phenotype relationship with biochemical representations of transcriptional and translational processes. This facilitates quantitative modelling of the relation between genome content, gene expression and cellular physiology. ( d ) When simulating cellular physiology, the transcriptional, translational and enzymatic activities are coupled to doubling time ( T d ) using constraints that limit transcription and translation rates as well as enzyme efficiency. τ mRNA , mRNA half-life; k cat , catalytic turnover constant; k translation , translation rate; ν , reaction flux. Full size image A modelling approach that accounts for the production and degradation of a cell's macromolecular machinery will provide a full genetic basis for every computed molecular phenotype ( Fig. 1b ). Such computations in turn enable the direct comparison of simulation to omics data and the simulation of variable expression and enzyme activity [13] , [14] . In other words, an integrated model of metabolism and macromolecular expression (ME-Model) affords a genetically consistent description of a self-propagating organism at the molecular level and moves us substantially closer to establishing a systems-level quantitative basis for biology. Here, we developed an ME-Modelling approach for the relatively simplistic microorganism, Thermotoga maritima , which metabolizes a variety of feedstocks into valuable products including H 2 (ref. 15 ). T . maritima possess a number of characteristics conducive to systems-level investigations of the genotype–phenotype relationship: a compact 1.8-Mb genome [16] , wealth of structural proteome data [17] , a limited repertoire of transcription factors (TFs) [18] and reduced genome organizational complexity compared with other microbes (H.L. et al ., Unpublished data). Taken together, T. maritima 's small set of TFs and reduced genome complexity impose a narrowed range of viable regulatory and functional states (H.L. et al ., unpublished data). The existence of few regulatory states may simplify the addition of synthetic capabilities and facilitate metabolic engineering efforts by reducing unexpected and irremediable side-effects arising from genetic manipulation [19] . A combination of metabolic versatility and genomic simplicity make T. maritima a promising candidate for investigating fundamental relationships between molecular and cellular physiology, both in silico and in vivo , and for the creation of a minimal chassis for chemical synthesis [20] . Our T. maritima ME-Model simulates changes in cellular composition with growth rate, in agreement with previously reported experimental findings [21] , [22] . We observed positive correlations between in silico and in vivo transcriptomes and proteomes for the 651 genes in our ME-Model with statistically significant ( P <1×10 −15 t -test) Pearson correlation coefficients (PCC) of 0.54 and 0.57, respectively. And, when we used our ME-Model as an exploratory platform for an in silico comparative transcriptomics study, we discovered putative TF-binding motifs and regulons associated with L -arabinose ( L -Arab) and cellobiose metabolism, and improved functional and transcription unit (TU) architecture annotation. Overall, ME-Models provide a chemically and genetically consistent description of an organism, thus they begin to bridge the gap currently separating molecular biology and cellular physiology. Genome-scale modelling of metabolism and expression We developed a network reconstruction and modelling method that includes macromolecular synthesis and post-transcriptional modifications in addition to metabolism ( Fig. 1c ; Supplementary Methods ). Specifically, our method accounts for the production of TUs, functional RNAs (that is, transfer RNAs (tRNAs), ribosomal RNAs (rRNAs) and so on) and peptide chains, as well as the assembly of multimeric proteins and dilution of macromolecules to daughter cells during growth. Based on available genomic, structural proteomic and biochemical literature we constructed an ME-Model for T. maritima that accounts for the functional activities of 50% of the annotated gene products and, more importantly, mechanistically links these enzyme activities to the genome. To accurately model self-replicating cells at the molecular level, it is necessary to account for material dilution during cell division as a result of volume doubling, and to provide limits on the number of proteins that may be translated from an messenger RNA before the mRNA decays or is transmitted to a daughter cell. To approximate dilution of transcripts and proteins to daughter cells and prevent infinite translation of peptides from an mRNA, we devised a series of coupling constraints ( Fig. 1d ; Supplementary Methods ). These constraints effectively provide upper limits on enzyme expression and activity and are a function of the organism's doubling time ( T d ). These coupling constraints may be tuned for specific mRNAs or enzymes if their, respective, degradation rates or catalytic turnover constants ( k cat ) are known. Applications of M-Models often involve simulating log-phase cellular growth using flux balance analysis (FBA) [23] , [24] . The organism's gross lipid, nucleotide, amino acid (AA) and cofactors, as well as growth-associated and maintenance ATP usage, are experimentally measured. Then, these measurements are integrated with the organism's T d to define a biomass reaction that approximates the dilution of cellular materials during formation of daughter cells. However, cellular composition is known to vary as a function of T d and medium [21] —with Schaechter et al . indicating that T d is more influential than growth medium. Our ME-Model explicitly describes transcription, translation and the dilution of gene products to daughter cells, thus it is unnecessary to use a gross biomass production reaction when simulating growth. Instead, ME-Models contain a structural reaction that accounts for the dilution of structural materials (that is, DNA, cell wall, lipids and so on) during division and the energy cost associated with cellular maintenance of the structure ( Supplementary Table S1 ). Conceptually, this structural reaction approximates the production of a cell whose composition varies as a function of environment and growth rate ( Fig. 2a ). 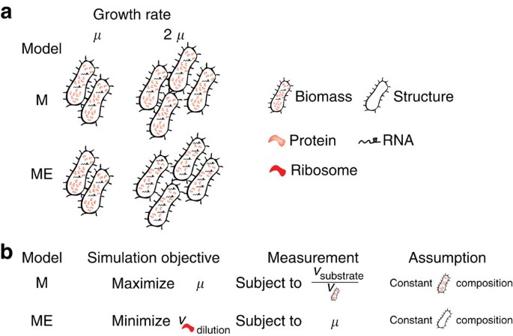Figure 2: Comparison of M- and ME-Models objective functions and assumptions. (a) M-Models simulate constant cellular composition (biomass) as a function of specific growth rate (μ), whereas ME-Models simulate constant structural composition with variable composition of proteins and transcripts. (b) Linear programming simulations with M-Models are designed to identify the maximumμthat is subject to experimentally measured substrate uptake rates. Only biomass yields are predicted asμenters indirectly as an input through the supplied substrate uptake rate (see the measurement column for M-Models). Importantly, the substrate uptake rate is derived by normalizing to biomass production. Linear programming simulations with ME-Models aim to identify the minimum ribosome production rate required to support an experimentally determinedμ.μenters into the coupling constraints and so it must be supplied (or sampled) as the problem would otherwise be a Nonlinear Program (NLP). As all M-Models reactions are contained within the ME-Models, ME-Models can simulate all M-Models objectives in addition to the broad range of objectives associated with macromolecular expression. Figure 2: Comparison of M- and ME-Models objective functions and assumptions. ( a ) M-Models simulate constant cellular composition (biomass) as a function of specific growth rate ( μ ), whereas ME-Models simulate constant structural composition with variable composition of proteins and transcripts. ( b ) Linear programming simulations with M-Models are designed to identify the maximum μ that is subject to experimentally measured substrate uptake rates. Only biomass yields are predicted as μ enters indirectly as an input through the supplied substrate uptake rate (see the measurement column for M-Models). Importantly, the substrate uptake rate is derived by normalizing to biomass production. Linear programming simulations with ME-Models aim to identify the minimum ribosome production rate required to support an experimentally determined μ . μ enters into the coupling constraints and so it must be supplied (or sampled) as the problem would otherwise be a Nonlinear Program (NLP). As all M-Models reactions are contained within the ME-Models, ME-Models can simulate all M-Models objectives in addition to the broad range of objectives associated with macromolecular expression. Full size image Molecularly efficient simulation of cellular physiology The RNA-to-protein mass ratio ( r ) has been observed to increase as a function of specific growth rate ( μ ) [21] , [22] and decreases as a function of translation efficiency [22] . Schaechter et al . also observed an increase in the number of ribonucleoprotein particles with increasing μ , whereas the translation rate per ribonucleoprotein particle was relatively constant [21] . The increase in r and ribonucleoproteins may be due to the reduced number of translation events mediated by a ribosome as T d decreases. To ascertain whether our ME-Model recapitulated the observed increases in r , ribosomal RNA and proteins with increasing μ , we simulated a range of growth rates in a defined minimal medium [25] ( Supplementary Table S2 ). To simulate the molecular physiology of T. maritima for a particular μ , we used FBA [24] subject to linear programming optimization [26] to identify the minimum ribosome production rate required to support a given μ ( Fig. 2b ). Ribosome production has been shown to be linearly correlated with growth rate in Escherichia coli [22] , [27] , [28] . Assuming that efficient use of enzymes contributes to the fitness of an evolutionarily adapted lineage [29] , we would expect a successful organism to produce the minimal amount of ribosomes required to support expression of the proteome. Consistent with experimental observations [21] , [22] , our ME-Model simulated an increase in r with increasing μ and with decreasing translation efficiency ( Fig. 3a ). We observed that the fraction of the transcriptome associated with ribosomal RNA in silico increased with μ ( Fig. 3b ). In addition, the ribosomal proteins account for a larger proportion of the total proteome as μ increases ( Fig. 3c ). These results indicate that it is possible to mechanistically model changes in cellular physiology that have only recently yielded to phenomenological modelling [22] . 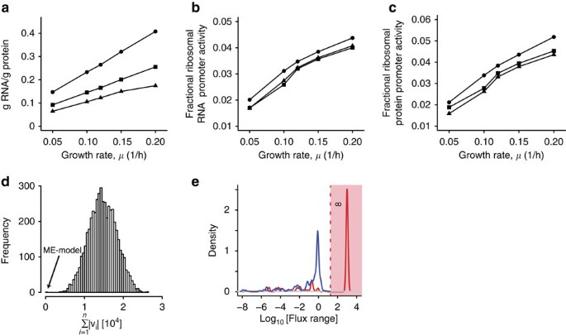Figure 3: Simulation of variable cellular composition and efficient use of enzymes. (a) With our ME-model, the RNA/protein ratio increases linearly with growth rate and with a slope proportional to translational capacity in amino acids per second (circles: 5 AA/s, squares: 10 AA/s, triangles: 20 AA/s). (b) Ribosomal RNA (rRNA) synthesis increases, relative to total RNA synthesis, with growth rate (symbols as ina). (c) Ribosomal protein promoter activity increases, relative to total RNA synthesis, with growth rate (symbols as ina). (d) Random sampling of the M-Model solution space indicates that the M-Model solution space contains numerous internal solutions with a broad range of total network flux. The probability of finding an M-Model solution as efficient as an ME-Model simulation is 2.1×10−5; the probability was calculated from a normal distribution constructed from the M-Model sample space. The M-Model sample contains 5,000 flux vectors randomly sampled from the M-Model solution space. (e) Smooth estimate of the density of the flux ranges for the metabolic enzymes that may be simulated while maintaining the objective for efficient growth with a 1% tolerance (M-Model: red line, ME-Model: blue line). The shaded area denotes biologically unrealistic flux values. All simulations were performed with anin silicominimal medium with maltose as the sole carbon source. Figure 3: Simulation of variable cellular composition and efficient use of enzymes. ( a ) With our ME-model, the RNA/protein ratio increases linearly with growth rate and with a slope proportional to translational capacity in amino acids per second (circles: 5 AA/s, squares: 10 AA/s, triangles: 20 AA/s). ( b ) Ribosomal RNA (rRNA) synthesis increases, relative to total RNA synthesis, with growth rate (symbols as in a ). ( c ) Ribosomal protein promoter activity increases, relative to total RNA synthesis, with growth rate (symbols as in a ). ( d ) Random sampling of the M-Model solution space indicates that the M-Model solution space contains numerous internal solutions with a broad range of total network flux. The probability of finding an M-Model solution as efficient as an ME-Model simulation is 2.1×10 −5 ; the probability was calculated from a normal distribution constructed from the M-Model sample space. The M-Model sample contains 5,000 flux vectors randomly sampled from the M-Model solution space. ( e ) Smooth estimate of the density of the flux ranges for the metabolic enzymes that may be simulated while maintaining the objective for efficient growth with a 1% tolerance (M-Model: red line, ME-Model: blue line). The shaded area denotes biologically unrealistic flux values. All simulations were performed with an in silico minimal medium with maltose as the sole carbon source. Full size image With M-Models, the cellular macromolecular composition is constant, ergo they cannot reproduce the observed increases in r or ribosomes with increasing μ . Although it is possible to empirically determine a relationship between gross biomass composition and μ and then use this relationship to study variable composition in M-Models [30] , the M-Models will compute a solution space where the range of activity for a number of enzymes may be rather broad and even infinite [7] , if not specifically constrained. The biologically implausible sections of the M-Model solution space are due, in large part, to unconstrained thermodynamically infeasible internal loops that can operate at an arbitrary flux level [8] . These arbitrary activities contradict previous observations that efficient organisms should maintain a minimal total flux through their biochemical network [29] , [31] . By explicitly accounting for enzyme expression and activity, ME-Model simulations should identify the set of proteins that will result in optimally efficient conversion of growth substrates into cells. To determine whether our ME-Model was more economic in terms of enzyme usage than the M-Model, we compared our ME-Model simulation to a random sampling of the M-Model solution space [7] . After we fit a normal distribution to the sampled M-Model space, we found that there is a small (2.1×10 −5 ) probability of finding an M-Model solution as efficient as the ME-Model solution ( Fig. 3d ). Because ME-Models explicitly account for the costs of enzyme expression and dilution to daughter cells, the most efficient growth simulations will minimize the materials required to assemble the cell; that is, ME-Models will efficiently use enzymes when simulating a μ . To compare the range of permissible, that is, computationally feasible, activity for each metabolic enzyme in the ME-Model versus the M-Model, we performed flux variability analysis. Flux variability analysis identifies the flux range that each reaction may carry given that the model must also simulate the specified objective value, such as μ , with a set tolerance. The permissible enzyme activities for simulating efficient growth with a 1% tolerance tended to have smaller ranges in the ME-Model compared with the M-Model ( Fig. 3e ; Supplementary Data 1 ), highlighting the sharply reduced flexibility in the ME-Model solution space when simulating optimal growth. Our ME-Model contains gene products that carry out 142 of the 206 functions estimated as essential for a minimal organism [32] , whereas the M-Model contains only 65 of these core functions. With the ME-Model, 120 of the 142 functions were essential for ribosome production, whereas only 23 of the 65 functions in the M-Model were essential for biomass production ( Supplementary Data 2 ). This broader coverage of cellular functions means that ME-Models may be used for in silico investigations of phenotypic states that are inaccessible to M-Models. Gene product production and turnover alters pathway activity In addition to simulating variable cellular composition and effectively eliminating the infinite catalysis problem, there are a number of metabolic activities that are required for optimally efficient growth with the ME-Model but not with the M-Model ( Fig. 4 ). These differences are due to the ME-Model producing small metabolites as by-products of gene expression and explicitly accounting for the material and energy costs of macromolecule production and turnover. The ME-Model includes metabolic activities for recycling S -adenosylhomocysteine, which is a by-product of rRNA and tRNA methylation, and guanine, which is a by-product of queuosine modification of various tRNAs ( Fig. 4a ). The ME-Model, also, produces CTP from CMP that is produced during mRNA degradation ( Fig. 4b ). Interestingly, the M-Model does not require CDP production to simulate growth, whereas CDP production is essential in the ME-Model. The ME-Model exhibits frugality with respect to central metabolic reactions ( Fig. 4c ) and proposes the canonical gylcolytic pathway during efficient growth, whereas the M-Model indicates that alternate pathways are as efficient. When the efficiency requirement is relaxed these less-efficient pathways may be active in the ME-Model solution space ( Supplementary Data 1 ). The genes associated with optimal activities tended to be strongly expressed (approximately 60th–90th percentile) in transcriptome data. 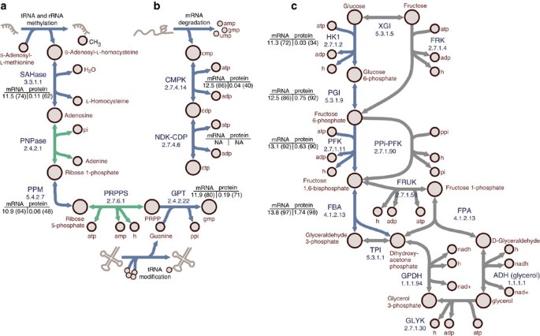Figure 4: Metabolic reactions required for efficient growth with the ME-Model but not the M-Model. (a) Recycling of by-products of RNA modifications. Adenosylhomocysteinease (SAHase) hydrolysesS-adenosylhomocysteine (SAH) toL-homocysteine (L-HCys) and adenosine. Purine nucleoside phosphorylase (PNP) phosphorylases adenosine to adenine and ribose-1-phosphate (Rib-1-P). Rib-1-P is converted to ribose-5-phosphate (Rib-5-P) by phosphopentomutase (PPM). Phosphoribosylpyrophosphate synthetase (PRPPS) phosphorylates Rib-5-P to produce 5-phosphoribosol-1-pyrophosphate (PRPP). Guanine phosphoribosyltransferase (GPT) produces GMP from the reaction of PRPP and guanine, which is a by-product of tRNA metabolism. (b) CMP produced during mRNA degradation is recycled to CTP using cytidylate kinase (CMPK) and nucleoside-diphosphate kinase (NDK-CDP). (c) The ME-model uses the canonical glycolytic pathway, whereas with the M-Model can circumvent portions during optimal growth simulations. The canonical pathway involves phosphorylation ofD-glucose (D-Glc) to glucose-6-phospate (G6P) by hexokinase (HK1). G6P is isomerized to fructose-6-phosphate (F6P) by phosphoglucose isomerase (PGI). F6P is phosphorylated to fructose-1,6-bisphosphate (FBP) by phosphofructokinase (PFK). FBP is metabolized to glyceraldehyde-3-phosphate (G3P) and dihydroxyacetone phosphate (DHAP) by FBP aldolase (FBA). The M-Model can circumvent the HK1/PGI portion with glucose/xylose isomerase (GXI) and fructokinase (FRK); however, HK1 or PGI must also be expressed because G6P is an essential metabolite. PFK can be circumvented by diphosphate-fructose-6-phosphate 1-phosphotransferase (PPi-PFK). FBA can be circumvented by a pathway using 1-phosphofructokinase (FRUK), fructose-1-phosphate aldolase (FPA), alcohol dehydrogenase (ADH(glycerol)), glycerol kinase (GLYK), glycerol-3-phosphate dehydrogenase (GPDH) and triose phosphate isomerase (TPI). Enzyme commission numbers are provided for each reaction. mRNA and protein expression (and quantile) values are provided. Flux variability analysis was performed for simulated growth on maltose minimal medium. Blue arrows: reactions required for optimally efficient growth with the ME-Model, but not the M-Model. Green arrows: active reactions in a single maltose minimal medium simulation shown to put results into pathway context. Grey arrows: alternate optimal pathways in the M-Model. Figure 4: Metabolic reactions required for efficient growth with the ME-Model but not the M-Model. ( a ) Recycling of by-products of RNA modifications. Adenosylhomocysteinease (SAHase) hydrolyses S -adenosylhomocysteine (SAH) to L -homocysteine ( L -HCys) and adenosine. Purine nucleoside phosphorylase (PNP) phosphorylases adenosine to adenine and ribose-1-phosphate (Rib-1-P). Rib-1-P is converted to ribose-5-phosphate (Rib-5-P) by phosphopentomutase (PPM). Phosphoribosylpyrophosphate synthetase (PRPPS) phosphorylates Rib-5-P to produce 5-phosphoribosol-1-pyrophosphate (PRPP). Guanine phosphoribosyltransferase (GPT) produces GMP from the reaction of PRPP and guanine, which is a by-product of tRNA metabolism. ( b ) CMP produced during mRNA degradation is recycled to CTP using cytidylate kinase (CMPK) and nucleoside-diphosphate kinase (NDK-CDP). ( c ) The ME-model uses the canonical glycolytic pathway, whereas with the M-Model can circumvent portions during optimal growth simulations. The canonical pathway involves phosphorylation of D -glucose ( D -Glc) to glucose-6-phospate (G6P) by hexokinase (HK1). G6P is isomerized to fructose-6-phosphate (F6P) by phosphoglucose isomerase (PGI). F6P is phosphorylated to fructose-1,6-bisphosphate (FBP) by phosphofructokinase (PFK). FBP is metabolized to glyceraldehyde-3-phosphate (G3P) and dihydroxyacetone phosphate (DHAP) by FBP aldolase (FBA). The M-Model can circumvent the HK1/PGI portion with glucose/xylose isomerase (GXI) and fructokinase (FRK); however, HK1 or PGI must also be expressed because G6P is an essential metabolite. PFK can be circumvented by diphosphate-fructose-6-phosphate 1-phosphotransferase (PPi-PFK). FBA can be circumvented by a pathway using 1-phosphofructokinase (FRUK), fructose-1-phosphate aldolase (FPA), alcohol dehydrogenase (ADH(glycerol)), glycerol kinase (GLYK), glycerol-3-phosphate dehydrogenase (GPDH) and triose phosphate isomerase (TPI). Enzyme commission numbers are provided for each reaction. mRNA and protein expression (and quantile) values are provided. Flux variability analysis was performed for simulated growth on maltose minimal medium. Blue arrows: reactions required for optimally efficient growth with the ME-Model, but not the M-Model. Green arrows: active reactions in a single maltose minimal medium simulation shown to put results into pathway context. Grey arrows: alternate optimal pathways in the M-Model. Full size image These differences highlight the interplay between macromolecular synthesis and degradation, metabolism and salvage, and optimal use of the proteome. The ME-Models allow a fine resolution view of these processes and their simultaneous reconciliation. Not only can one analyse specific pathways in isolation, such as the three examples given above, but it is now possible to investigate in detail the coordination of functions within an organism's biochemical repertoire. Simulation of systems-level molecular phenotypes To assess our ME-Model's ability to simulate systems-level molecular phenotypes, we compared model predictions to substrate consumption, product secretion, AA composition, transcriptome and proteome measurements. With the only external constraints for the ME-Model being the experimentally determined μ during log-phase growth in maltose minimal medium at 80 °C, our model accurately predicted maltose consumption and acetate and H 2 secretion ( Fig. 5a ; Supplementary Table S3 ). Predicted AA incorporation was linearly correlated (0.79 PCC; P <4.1×10 −5 t -test) with measured AA composition ( Fig. 5b ). 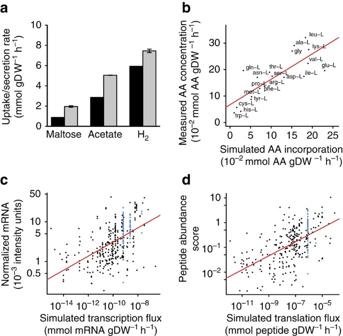Figure 5: The ME-Model accurately simulates molecular phenotypes during log-phase growth. (a) The ME-Model accurately simulates H2and acetate secretion with maltose uptake when constrained with a measured growth rate (n=2). Experiment: grey bars, simulation: black bars. (b) Thein silicoribosome incorporates the 20 amino acids at rates proportional (Pearson correlation coefficient=0.79;P< 4.1×10−5t-test) to the bulk amino-acid composition of aT. maritimacell as measured by high-performance liquid chromatography (n=1). (c) Simulated transcriptome fluxes are significantly (P<2.2×10−16t-test) and positively correlated (Pearson correlation coefficient=0.54) with semiquantitativein vivotranscriptome measurements (n=4). RNAs containing ribosomal proteins (blue) were expressed stoichiometrically in simulations but exhibited variability in measurements. (d) Simulated translation fluxes are significantly (P<2.2×10−16t-test) and positively correlated (Pearson correlation coefficient=0.57) with semiquantitativein vivoproteomic measurements (n=3). Ribosomal proteins (blue) were expressed stoichiometrically in simulations but exhibited variability in measurements. Figure 5: The ME-Model accurately simulates molecular phenotypes during log-phase growth. ( a ) The ME-Model accurately simulates H 2 and acetate secretion with maltose uptake when constrained with a measured growth rate ( n =2). Experiment: grey bars, simulation: black bars. ( b ) The in silico ribosome incorporates the 20 amino acids at rates proportional (Pearson correlation coefficient=0.79; P < 4.1×10 −5 t -test) to the bulk amino-acid composition of a T. maritima cell as measured by high-performance liquid chromatography ( n =1). ( c ) Simulated transcriptome fluxes are significantly ( P <2.2×10 −16 t -test) and positively correlated (Pearson correlation coefficient=0.54) with semiquantitative in vivo transcriptome measurements ( n =4). RNAs containing ribosomal proteins (blue) were expressed stoichiometrically in simulations but exhibited variability in measurements. ( d ) Simulated translation fluxes are significantly ( P <2.2×10 −16 t -test) and positively correlated (Pearson correlation coefficient=0.57) with semiquantitative in vivo proteomic measurements ( n =3). Ribosomal proteins (blue) were expressed stoichiometrically in simulations but exhibited variability in measurements. Full size image FBA simulates reaction fluxes, whereas transcriptomics and proteomics technologies provide semiquantitative measurements of expressed gene product abundance. Thus, the simulated fluxes through the transcriptome and proteome do not directly approximate the respective omics measurements; however, for macromolecules there should be a positive correlation between gene and protein synthesis fluxes and the respective gene product abundances during log-phase growth. In other words, proteins and genes are relatively stable and when an organism is growing at steady state a relative increase in expression rate for a protein will effectively increase the quantity of that protein. Interestingly, when we compared the simulated transcriptome and proteome fluxes to transcriptome and proteome measurements, respectively, there were statistically significant ( P <2.2×10 −16 t -test) positive correlations for both the transcriptome (0.54 PCC; Fig. 5c ) and the proteome (0.57 PCC; Fig. 5d ). This degree of concordance was unexpected because the model does not account for transcriptional regulation or transcript-specific RNA degradation rates. However, this concordance may be the result of our simulation objective being aligned with T. maritima 's regulatory programme, whereas a decreased concordance would be expected if the regulatory network was responding to a stress. We have previously observed a tendency to increase the expression of metabolically efficient pathways, and decrease inefficient alternatives, by E. coli after adaptive evolution under growth selection pressure [31] . Also, we have observed that T. maritima 's genome is highly active with >89% of the protein-coding genes expressed in diverse conditions (H.L. et al ., Unpublished data), which could indicate a general eschewal of complex and expensive circuitry within the global regulatory strategy. Approximately 30% of T. maritima 's genome is not functionally annotated and 50% of the functionally annotated genes fall outside of the scope of our ME-Model. A number of genes not accounted in our model were expressed in vivo ( Supplementary Fig. S1 ), and the costs of their expression as well as their functional activities may contribute to the differences between simulation and measurement. In addition, unknown regulatory features might be responsible for irregularities observed when comparing simulation to the measurement. For instance, ribosomal RNAs and proteins are expected to be expressed at stoichiometric ratios, as occurs with the simulation, yet there is sizable variability in their measured values ( Fig. 5c,d , blue colouring). These results illustrate that it is possible to sketch a molecular description of a replicating organism solely from simple, but stoichiometrically accurate, chemical equations represented on a genome scale. In silico gene expression profiling drives discovery With our ME-Model it is now possible to compute the gene expression profile associated with growth in a specific condition or for a specific mutant. These gene expression profiles may then be compared to identify genes that are likely differentially regulated. The set of differentially expressed in silico genes may then be used to drive biological discovery or improve our model ( Fig. 6 ). 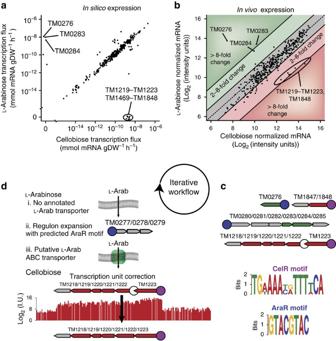Figure 6:In silicotranscriptome profiling drives biological discovery. (a)In silicocomparative transcriptomics identifies sets of genes that are differentially regulated for growth inL-arabinose (L-Arab) versus growth in cellobiose minimal media. TM0276, TM0283 and TM0284 are essential for metabolizingL-Arab, whereas TM1219–TM1223, TM1469 and TM1848 are essential for metabolizing cellobiose. (b)In vivotranscriptome measurements (n=2) confirm thein silicotranscriptomics predictions for differential expression of genes when metabolizingL-Arab or cellobiose. (c) Two distinct putative TF-binding motifs are present upstream of the TUs containing genes differentially expressedin silicowhen simulating growth inL-Arab versus cellobiose minimal media. The motif upstream of the genes upregulated during growth inL-Arab medium is termed AraR, whereas the motif of the genes upregulated during growth in cellobiose medium is termed CelR. Genes (grey: not in the model, green: upregulated byL-arabinose, red: upregulated by cellobiose) organized into TUs involved in the shift are shown. Each TU contains a promoter region (circle) arbitrarily taken to be 75 base pairs upstream of the first gene in the TU. Promoters found to contain the AraR or CelR motifs are coloured blue and purple, respectively. (d) SearchingT. maritima's genome for additional AraR and CelR motifs results in new biological knowledge. AlthoughT. maritimacan metabolizeL-Arab, there is no annotated transporter in the current genome. We identified a putative AraR motif in a single TU (TM0277/0278/0279) not contained in the ME-Model. Analysis of the TM0277/0278/0279 TU with the SEED RAST server indicated that the genes are likely components of an ABC transporter that may be associated withL-Arab transport. The CelR motif was not present in the promoter region upstream of the cellobiose transporter operon (TM1218/1219/1220/1221/1222); however, the CelR motif was present in the promoter of the TU (TM1223) directly upstream of the cellobiose transport operon. Examination of thein vivotranscriptome measurement indicates that the cellobiose transporter operon belongs to the same TU as that of TM1223. Figure 6: In silico transcriptome profiling drives biological discovery. ( a ) In silico comparative transcriptomics identifies sets of genes that are differentially regulated for growth in L -arabinose ( L -Arab) versus growth in cellobiose minimal media. TM0276, TM0283 and TM0284 are essential for metabolizing L -Arab, whereas TM1219–TM1223, TM1469 and TM1848 are essential for metabolizing cellobiose. ( b ) In vivo transcriptome measurements ( n =2) confirm the in silico transcriptomics predictions for differential expression of genes when metabolizing L -Arab or cellobiose. ( c ) Two distinct putative TF-binding motifs are present upstream of the TUs containing genes differentially expressed in silico when simulating growth in L -Arab versus cellobiose minimal media. The motif upstream of the genes upregulated during growth in L -Arab medium is termed AraR, whereas the motif of the genes upregulated during growth in cellobiose medium is termed CelR. Genes (grey: not in the model, green: upregulated by L -arabinose, red: upregulated by cellobiose) organized into TUs involved in the shift are shown. Each TU contains a promoter region (circle) arbitrarily taken to be 75 base pairs upstream of the first gene in the TU. Promoters found to contain the AraR or CelR motifs are coloured blue and purple, respectively. ( d ) Searching T. maritima 's genome for additional AraR and CelR motifs results in new biological knowledge. Although T. maritima can metabolize L -Arab, there is no annotated transporter in the current genome. We identified a putative AraR motif in a single TU (TM0277/0278/0279) not contained in the ME-Model. Analysis of the TM0277/0278/0279 TU with the SEED RAST server indicated that the genes are likely components of an ABC transporter that may be associated with L -Arab transport. The CelR motif was not present in the promoter region upstream of the cellobiose transporter operon (TM1218/1219/1220/1221/1222); however, the CelR motif was present in the promoter of the TU (TM1223) directly upstream of the cellobiose transport operon. Examination of the in vivo transcriptome measurement indicates that the cellobiose transporter operon belongs to the same TU as that of TM1223. Full size image Towards this end, we computed the transcriptome profiles for T. maritima grown in a minimal medium with either L -Arab or cellobiose as the sole carbon source ( Fig. 6a ). Our computations identified genes that were exclusively expressed and essential for growth with each carbon source. Because these genes are essential for growth on the respective substrate they are conditionally essential genes. Conditionally essential genes are often subject to transcriptional regulation, however, they may be constitutively expressed. To assess whether the genes were differentially expressed in vivo , we measured the transcriptome of T. maritima growing in minimal medium with L -Arab or cellobiose as the carbon source. The genes with the strongest differential expression in vivo were among the set of differentially expressed genes in silico ( Fig. 6b ) providing supporting evidence for the presence of transcriptional regulation. Conditionally expressed genes may be regulated by the same TF [33] . The presence of a common motif in the promoter regions of a set of genes may indicate regulation by a common TF. To identify potential TF-binding motifs, we scanned the promoter and upstream regions of the in silico differentially expressed genes with MEME (Multiple Expectation Maximum for Motif Elicitation) [34] . Surprisingly, there was a high-scoring motif for the genes essential for growth on L -Arab and a high-scoring motif for the genes essential for growth on cellobiose ( Fig. 6c ). The motif found upstream of the L -Arab upregulated genes is similar to the AraR motif from Bacillus subtilis [35] ( Supplementary Fig. S2 ). Also, the motif upstream of the cellobiose upregulated genes bears resemblance to catabolite-responsive elements ( cres ), known to have an important global role in catabolite repression through the binding of the CcpA protein in B. subtilis [36] . Here, we term the motif the CelR motif, as the regulated genes are involved in cellobiose metabolism. These discoveries highlight how ME-Model simulations can guide discovery of new regulons. After identifying the putative AraR and CelR motifs, we scanned T. maritima' s genome for the presence of other members of the putative regulons. For the nondegenerate AraR motif 5′-GTACGTAC-3′, we identified a single additional instance in an intergenic region upstream of the TU-containing genes TM0277, TM0278 and TM0279 ( Fig. 6d ). These genes were induced when L -Arab was the carbon source, but not when cellobiose or maltose serves as the carbon source ( Supplementary Fig. S3 ). L -Arab transport is an orphaned activity in our model, which means that T. maritima may import L -Arab, however, the responsible loci are not known. When we examined these genes using the SEED RAST server [37] , TM0278 and TM0279 were classified as permeases of an ABC transporter putatively involved in L -Arab utilization, whereas TM0277 was not classified because it was annotated as containing an authentic frameshift [38] . Recent resequencing of T. maritima 's genome (H.L. et al ., Unpublished data) refute the initial annotation that TM0277 contains a frameshift mutation; and the SEED RAST annotation for TM0277 is a predicted sugar-binding protein for an arabinoside ABC transporter. Interestingly, the TUs containing ABC transporters for maltose and chitobiose are organized in the same manner: a binding protein followed by two permeases. The presence of the AraR motif, the strong upregulation of the TM0277/TM0278/TM0279 TU in response to L -Arab in vivo , the SEED RAST classification and resequenced genome strongly suggest that we have identified a functional L -Arab transport system in this organism. This discovery illustrates how in silico molecular biology at the genome scale can be used to expand regulons and improve genome annotation. When we scanned T. maritima 's genome for matches to the degenerate CelR motif TGWAAAYRTTTWCA, the promoter regions of TUs associated with cellobiose metabolism were identified. Interestingly, the promoter region of the TU-containing TM1222, TM1221, TM1220, TM1219 and TM1218 did not contain a CelR motif ( Fig. 6c,d ). TM1222, TM1221, TM1220 and TM1219 encode for a cellobiose ABC transporter, while TM1218 is annotated as a LacI family transcription regulator. However, the promoter region of the TU for TM1233, which is directly upstream of TM1222, contains the CelR motif. TM1233 encodes for the cellobiose-binding protein that facilitates cellobiose transport. In the TU architecture of our model, there was a predicted Rho-independent terminator following TM1223 that resulted in a new TU starting with TM1222. However, no promoter was detected in the intergenic region between TM1223 and TM1222 using PromBase [39] . This result leads us to believe that the initial assignment of TM1223 and TM1222 to separate TUs was incorrect ( Fig. 6d ). The presence of the cellobiose transport system in the updated TU, the strong CelR motif and the annotation of TM1218 as a TF suggest that TM1218 may encode for CelR. Our ME-Modelling approach represents a fundamental advance in the evolution of genome-scale biochemical models of life and significantly broadens the scope of microbial systems biology. It is now possible to ask systems-level questions in silico beyond metabolism and quantitatively analyse, in a bottom-up and mechanistic manner, a variety of omics data in the context of a growing organism. For instance, we can use a systems perspective to identify the minimal number of genes required to support homeostasis and replication—120 of the 142 of the proposed minimal bacterial genome [32] were essential for ribosome production in maltose minimal medium ( Supplementary Data 2 ). Not only can ME-Models predict global phenotypes that are traditionally employed with M-Models, such as maximal growth rate in a defined medium, but they can also be used to calculate whether the system has any material and energy reserves available for ancillary functions. For example, the measured maltose consumption rate was greater than the one that we calculated for economically efficient growth ( Fig. 5a ). This discrepancy between measurement and simulation could indicate that T. maritima does not strive for economic efficiency or represent the portion of sugar used to support the activities of the unannotated genes or regulatory circuitry. Given that the expression levels for the gene products associated with the more efficient pathways were highly expressed ( Fig. 4c ), we are disposed towards the latter. Although the ME-Model does not account for regulatory events, the presence of a strong discordance between simulation and measurement would indicate that factors other than economic efficiency are influencing the expressome, thus informing hypothesis generation. For example, if a more expensive isozyme was expressed in vivo than in silico , then it would be possible to estimate the improvement in k cat required for the expensive isozyme to offset its higher materials and energy costs. Technological advances have contributed to an expanding ocean of omics data that has been under-explored [3] . Omics data have been under-analysed, in part, due to the lack of a mechanistic systems-level framework for analysing myriad molecular components in the context of cellular physiology. To date, with the notable exception of C13 metabolic flux analysis, it has only been possible to perform indirect comparative analysis between omics data and M-Models [31] or to neglect the complexity of the genotype–phenotype relationship and use omics data as ad hoc constraints for M-Model enzyme activities [9] , [10] , [11] , [12] . Because ME-Models explicitly represent gene expression, directly investigating omics data in the context of the whole is now feasible. Viewing multi-omics data in the context of biochemically and genomically consistent ME-Models may allow us to extract more value from legacy and future omics data. Comparing in silico and in vitro transcriptomes, or proteomes, can highlight under-explored areas of molecular biology. For example, a set of genes highly expressed in silico but not expressed in vivo may indicate the presence of transcriptional regulation. Differential expression of a class of genes may indicate incompleteness in our knowledge of how those gene products interact or allude to, heretofore unknown, moonlighting functions. For instance, in the case of ribosomal proteins ( Fig. 5c,d , blue) the model predicts uniform expression, whereas omics measurements exhibit variability. The model was designed based on evidence that ribosomal protein synthesis is highly coordinated [40] , and does not account for feedback circuits affecting degradation rates that have yet to be fully elucidated [40] , [41] . Although there is a positive correlation between the simulated transcriptome fluxes and semiquantitative transcriptome data there was still a substantial amount of dispersion ( Fig. 5c ). When comparing in silico and in vivo transcriptome measurements it is important to realize that both are approximations of the transcript levels in an organism, and that omics technologies have been inherently noisy to date [42] . Incomplete knowledge, such as a lack of specific translation efficacy for each protein and degradation rates for each mRNA, and lack of signalling and regulatory circuitry will contribute to deviations from reality by ME-Model simulations. Similarly, probe-binding and sample-labelling efficacies, as well as other technical issues, serve as barriers to absolute quantitative transcriptome measurements [43] . Although it is a non-trivial endeavour to identify the source of all variation between the simulated and measured transcriptomes, it is possible to use the ME-Model for comparative transcriptomics approaches similar to two-channel DNA microarray studies. Despite the early technological limitations of DNA microarrays, biological discovery was enabled by performing comparative transcriptomics [44] , [45] , [46] , [47] . Transcriptome profiling has been used extensively to identify genes that are differentially regulated as a function of genetics and environment [44] . Analysis of differentially expressed genes has contributed to the identification of gene products responsible for unannotated enzymatic activities [45] . In combination with sequence analysis, differential gene expression data can be used to investigate transcriptional regulation [46] , [47] . We devised and implemented a workflow for in silico comparative transcriptomics, which resulted in the discovery of new regulons and improved both genome and TU annotation ( Fig. 6a–d ). The similarities between the comparative transcriptomics in silico ( Fig. 6a ) and in vivo ( Fig. 6b ) studies are striking, given the variation observed between the simulated and measured transcriptomes ( Fig. 5c )—this emphasizes that, in spite of its shortcomings, the ME-Modelling framework is a powerful tool for biological research. Finally, ME-Models enable integrated molecular biology on a genome scale while accounting for the metabolic requirements, which partially fulfills the challenge of Project K [48] and moves us one step closer to a molecular representation of CellMap [1] . Network reconstruction procedure The detailed procedure and formalism are described in detail in the Supplementary Methods . Our method accounts for biochemical reactions associated with transcription of TUs, TU degradation, translation, protein maturation, RNA processing, protein complex formation, ribosomal assembly, rRNA modification, tRNA modification, tRNA charging, aminoacyl-tRNA synthetase charging, charging EF-Tu, cleavage of polycistronic TUs to release stable RNA products, sources, sinks and tRNA activation (EF-TU) as well as metabolism. In our formalism, metabolic reactions are represented as multi-step processes including substrate binding by the enzyme and dissociation of substrate–enzyme complex to enzyme and products. The metabolic content for our reconstruction was based on the previously published model [17] , with updates to correct errors and incorporate new data ( Supplementary Data 3 ). The molecular machinery (for example, proteins, genes, RNAs) involved in macromolecular synthesis were identified from the genome annotation [16] , SEED subsystem analysis [49] , comparative genomics analysis of the E. coli model [28] and KEGG [38] . The functions of each of the 159 proteins associated with macromolecular synthesis in T. maritima were determined by primary literature when available. When no primary literature was available, the Uniprot [50] and SEED [49] databases were used to infer function by homology. All proteins currently believed to be used for macromolecular synthesis by T. maritima are enumerated in Supplementary Data 4 , and 93% of these genes are mechanistically linked in our ME-Model. The reactions associated with transcription and translation, including initiation, biopolymerization and termination, were generated from the genome sequence and a set of T. maritima template reactions ( Supplementary Methods ). In our modelling formalism, reversible reactions were represented as two unique reactions: one for the forward direction and one for the reverse. Protein complexes For each functional protein, we used primary literature and the RCSB Protein Data Bank [51] to determine whether the machine was a monomer or oligomer. The Protein Data Bank entries provided an opportunity to integrate 3D structural data into our reconstruction (this model includes structures for 32 additional open reading frames compared with Zhang et al . ). When data for multimeric state were unavailable for a protein of interest, state data for orthologs from closely related organisms were used; otherwise, the Uniprot database [50] was consulted. In the absence of data providing insight into the multimeric state of the protein, we assumed that the functional protein was a monomer. Genetic code determination From inspection of tRNA sequences and structures downloaded from the transfer RNA database [52] , we determined that T. maritima uses uniform-GUC decoding with only 46 tRNA genes (see Supplementary Data 5 ). In both Archaea and Bacteria, but not in Eukarya, the conversion of C34 of a CAU-anticodon to lysidine (k2C) or analogue generates an anticodon for isoleucine [53] . TMtRNA-Met-2 was assigned this role based on a strong sequence alignment to E. coli tRNAs containing k2C. The T. maritima genome encodes two additional tRNA genes with CAU anticodons, TMtRNA-Met-1 and TMtRNA-Met-3. Based on structural similarity [54] to those found in a crystal structure of E. coli 's formyl-methionyl-tRNAfMet [55] , TMtRNA-Met-1 may be involved in translation initiation, therefore, TMtRNA-Met-3 was designated to participate in translation elongation. TU architecture determination We assembled a draft TU architecture ( Supplementary Data 6 ) for T. maritim a based on a series of rules ( Supplementary Methods ). In short, we assumed all TUs start with a gene start and proceed until one of the following conditions is met: (1) two genes are found in convergent orientation on different strands, (2) two genes are found in divergent orientation on different strands, (3) a high-confidence Rho-independent transcription terminator is found separating two genes oriented in series on the same strand, (4) more than 55 base pairs separate two genes in series on the same strand or (5) experimental evidence indicates a TU boundary. Finally, to reflect the possibility of internal transcription start sites in TUs reconstructed using the rules above, we added an additional TU in cases where a high-confidence promoter was found in the region separating two genes oriented in series on the same strand. In silico molecular biology Log-phase growth simulations were performed using FBA [24] . Linear programming was used to identify the maximum μ or minimum ribosome production flux supporting a particular μ from the components of the in silico minimal media. Because of the presence of fast (metabolic) and slow (macromolecular synthesis) timescale reactions, the parameters in the ME-Model span a wide range that can result in inaccurate simulations due to floating point limitations of currently available floating point linear programming software ( Supplementary Methods ). To remove the possibility of simulation results being artefacts arising from floating point limitations, we used the exact simplex routines available in the QSopt_ex package [26] , with default parameter settings for ME-Model simulations. The predicted transcription level of a gene was determined by summing across the sink fluxes of TUs containing the gene, which is equivalent to the transcription fluxes less the TU degradation fluxes. Translation levels were reported as the sum across the relevant translation initiation fluxes, as many TUs can contribute to the production of a given protein. These values were compared with each other in the case of simulated nutrient shifts or to the abundances reported experimentally. In vivo methods T. maritima MSB8 (ATCC: 43589) was grown in 500 ml serum bottles containing 200 ml of anoxic minimal media with 10 mM maltose, L -arabinose or cellobiose as the sole carbon source at 80 °C. All samples were collected during log-phase growth. Substrate uptake and by-product secretion rates, compositional analyses, and transcriptome and proteome measurements were performed as described in the Supplementary Methods . Transcriptome data have been submitted to the NCBI Gene Expression Omnibus (accession ID: GSE28822 ) and processed values are in Supplementary Data 7 . Proteomics data are available through Pacific Northwest National Laboratory ( http://omics.pnl.gov ) and processed values are in Supplementary Data 8 . RNA modifications A variety of post-transcriptional modifications of rRNAs are represented in our model. For 16S rRNA, there was experimental evidence for ten modifications [56] in this organism ( Supplementary Table S4 ). The locations of pseudouridines, which are mass silent, were not available, but an 11th modification, U to Y at position 516, was included in the reconstruction based on the fact that it is well conserved in bacteria and the alignment ( Supplementary Data 9 ) supports its inclusion. An unusual derivative of cytidine-designated N-330 has been sequenced to position 1,404 (ref. 56 ) in the decoding region of the 16S rRNA. This modified nucleoside was excluded from the reconstruction as the exact chemical composition of the modification is unknown. We were unable to find organism-specific literature supporting modifications to the 5S and the 23S rRNA. Modifications to 5S rRNA are infrequent in bacteria [57] . Attempting to extrapolate 23S rRNA modifications from E. coli was relatively unsuccessful as alignment via ClustalW2 [58] showed significant differences near many of the putative modification sites ( Supplementary Data 10 ). The alignment reveals that the 23S rRNA of T. maritima is significantly longer (>100 bp) than that of E. coli . Only three proteins with annotated roles in modifying the 23S rRNA were added to the model for a total of six modifications ( Supplementary Table S5 ). Those were TM0940, TM0462 and TM1715. Post-transcriptional modification of tRNA also requires a significant investment in genes, enzymes, substrates and energy [59] . We included a variety of modifications ( Supplementary Table S6 ) in our model based on bioinformatics predictions and literature evidence ( Supplementary Table S7 ). Sensitivity analysis To explore the influence of some of the newly introduced parameters on model output, the bulk parameters used for the coupling constraints ( Supplementary Methods ) were varied (two-, four- and eight-fold increases and decreases away from the parameter set used). The results are summarized in Supplementary Fig. S4 . File formats Our final model is available as a Systems Biology Markup Language (SBML) XML file ( Supplementary Data 11 ). The model is also available as an LP file ( Supplementary Data 12 ) for use with linear programming solvers. Accession codes: Transcriptome data have been submitted to the NCBI Gene Expression Omnibus under accession code GSE28822 . How to cite this article: Lerman, J.A. et al . In silico method for modelling metabolism and gene product expression at genome scale. Nat. Commun. 3:929 doi: 10.1038/ncomms1928 (2012).